Inactivation of the Hippo tumour suppressor pathway by integrin-linked kinase One of the hallmarks of cancers is the silencing of tumour suppressor genes and pathways. The Hippo tumour suppressor pathway is inactivated in many types of cancers, leading to tumour progression and metastasis. However, the mechanisms of pathway inactivation in tumours remain unclear. Here we demonstrate that integrin-linked kinase (ILK) plays a critical role in the suppression of the Hippo pathway via phospho-inhibition of MYPT1-PP1, leading to inactivation of Merlin. Inhibition of ILK in breast, prostate and colon tumour cells results in the activation of the Hippo pathway components MST1 and LATS1 with concomitant inactivation of YAP/TAZ (Yes-associated protein/transcriptional co-activator with PDZ-binding motif) transcriptional co-activators and TEAD-mediated transcription. Genetic deletion of ILK suppresses ErbB2-driven YAP/TAZ activation in mammary tumours, and its pharmacological inhibition suppresses YAP activation and tumour growth in vivo . Our data demonstrate a role for ILK as a multiple receptor proximal regulator of Hippo tumour suppressor pathway and as a cancer therapeutic target. Tumour progression, metastatic potential and response to therapy depend on complex genetic, epigenetic and tumour microenvironmental interplay. Despite intensive efforts at identifying genetic mutations that promote tumour progression, genetically identical tumour cells have been demonstrated to behave very differently in vivo [1] , [2] . The bidirectional interaction between tumour cells and the tumour microenvironment can influence the tumour phenotype by switching intracellular signalling pathways on or off, or by switching from one signalling pathway to another [3] , [4] , thus evading the effects of therapeutics and promoting tumour recurrence and metastasis. The highly evolutionarily conserved Hippo tumour suppressor signalling pathway [5] , [6] , which restricts organ size and proliferation, has emerged as one such prominent pathway which is ‘switched off’ in many types of cancers. Core components of the Hippo pathway include the mammalian sterile 20-like kinases (MSTs), Large tumour suppressor kinases (LATSs) and the adaptor proteins Salvador homologue 1 (SAV1; also called WW45) and Mps One Binder kinase activator proteins [7] . The major target of the Hippo core kinase cascade is the mammalian transcriptional activator Yes-associated protein (YAP) and its paralogue transcriptional co-activator with PDZ-binding motif (TAZ). Phosphorylation of YAP and TAZ by the Hippo pathway leads to their sequestration in the cytoplasm by interaction with 14-3-3 proteins and ubiquitination-dependent proteosomal degradation [8] . In cancer, Hippo signalling is inactivated, and YAP and TAZ are activated and free to translocate into the nucleus to promote cell proliferation. Nuclear YAP/TAZ activate or suppress transcription factors that regulate target genes involved in cell proliferation, tissue growth, control of organ size and shape or metastasis [5] , [9] , [10] , [11] , [12] . These transcription factors include: TEAD1–4 (important for growth promotion and epithelial–mesenchymal transition), SMADs (TGF-β (transforming growth factor beta) signalling), RUNXs (blood and bone formation), p63/p73 (apoptosis), PAX3 (neural crest formation), PPARc (adipogenesis), TTF1 (thyroid and lung morphogenesis) and TBX-5 (WNT/β-catenin signalling and cardiac and limb development) [7] . Although recent reports have identified upstream positive and negative regulators of the pathway [10] , [13] , its membrane proximal components are not established, although cell density and actin cytoskeletal organization can modulate the pathway [14] , [15] . Integrin-linked kinase (ILK) is an integrin associated, actin and tubulin cytoskeletal interacting effector, which regulates several cell adhesion and integrin-mediated as well as growth factor-regulated functions [16] , [17] , [18] . ILK coordinates several signalling pathways, and it has been shown to activate Pi3Kinase/Akt, Wnt, TGF-β and epithelial–mesenchymal transition signalling in various types of cancer cells [16] , [17] . Furthermore, ILK expression is upregulated in many types of cancers [17] , [18] . We therefore wanted to determine whether ILK signalling cross-talks with the Hippo pathway. Here we demonstrate that ILK is a critical negative regulator of the Hippo tumour suppressor pathway in human breast, prostate and colon cancer cells. ILK, by inhibiting MYPT1 through direct phosphorylation, prevents Merlin dephosphorylation and activation, resulting in the inhibition of the Hippo kinase cassette and nuclear accumulation of YAP/TAZ. Inhibition of ILK expression with siRNA or pharmacological inhibition of its activity, results in a dramatic activation of the Hippo pathway, leading to YAP/TAZ phosphorylation and sequestration in the cytoplasm, with concomitant inhibition of TEAD transcriptional activity. Furthermore, genetic knockout of ILK in ErbB2-activated mammary tumours leads to YAP inactivation, as does pharmacological inhibition of breast tumour growth in xenograft tumour models in vivo . These data collectively point to an important role of ILK in inhibiting the Hippo tumour suppressor pathway in cancer cells, and identifying ILK as a potential therapeutic target for re-activation of Hippo signalling. Inhibition of ILK leads to YAP inactivation in tumour cells Hippo pathway perturbation can trigger tumorigenesis in mice, and mutations and altered expression of a subset of Hippo pathway genes have been observed in human cancers [19] , [20] . To determine a potential role of ILK in the suppression of the Hippo pathway, we initially examined the phosphorylation status of YAP protein in different human tumour cell lines. As shown in Fig. 1a , we found that phosphorylation of YAP on Ser127 was significantly enhanced upon siRNA-mediated knockdown of ILK expression in HCT116 colon and PC3 prostate tumour cells, indicating that inhibition of ILK leads to YAP inactivation in these cell lines. In addition, we utilize MDA-MB-435 LCC6 breast cancer cells to examine as well YAP/TAZ nucleo/cytoplasmic localization in response to ILK depletion. As shown in Fig. 1b , extensive localization of YAP is shown in the nuclei of MDA-MB-435 LCC6 breast cancer cells, which was sequestered to the cytoplasm in ILK siRNA-treated cells. These data suggest that in these human colon, prostate and breast cancer cell lines, the Hippo pathway is inactivated and that ILK plays a role in this inactivation since inhibition of ILK expression resulted in the phosphorylation of YAP and its sequestration in the cytoplasm. 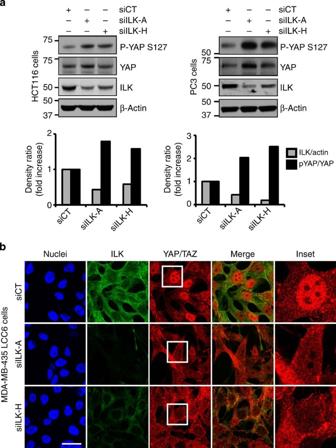Figure 1: Silencing ILK leads to functional inactivation of YAP/TAZ in cancer cells. Indicated cells were treated with non-silencing control (siCT) or two different siRNAs against ILK (siILK-A or siILK-H): (a) Cell lysates were subjected to western blotting with the indicated antibodies. Bands were semiquantified by image intensity area under the curve. (b) Cells were subjected to immunofluorescence microscopy with the indicated antibodies. Scale bar, 20 μm. Figure 1: Silencing ILK leads to functional inactivation of YAP/TAZ in cancer cells. Indicated cells were treated with non-silencing control (siCT) or two different siRNAs against ILK (siILK-A or siILK-H): ( a ) Cell lysates were subjected to western blotting with the indicated antibodies. Bands were semiquantified by image intensity area under the curve. ( b ) Cells were subjected to immunofluorescence microscopy with the indicated antibodies. Scale bar, 20 μm. Full size image To examine the role of ILK in regulating the pathway in more detail, we treated PC3 and HCT116 human tumour cells with a highly specific inhibitor of ILK kinase activity [16] , [18] , [21] . This small molecule inhibitor, QLT0267, has previously been tested against 150 protein kinases and found to be highly selective at inhibiting ILK activity relative to other kinases [21] with only one off-target kinase reported, the FMS-like tyrosine kinase 3 (ref. 22) [22] . As shown in Fig. 2a , treatment of these cell types, under standard growth conditions, with 10 μ M QLT0267 resulted in a time-dependent stimulation of phosphorylation of MST1 (T183), LATS1 (T1079) and YAP (S127). In addition, since phosphorylated YAP and TAZ have been demonstrated to be sequestered in the cytoplasm by 14.3.3 (ref. 8) [8] , we observed that in both cell lines, inhibition of ILK resulted in the sequestration of YAP to the cytoplasm with partial 14:3:3 co-localization, compared with cells treated with dimethylsulphoxide (DMSO) (vehicle), in which YAP was almost exclusively localized to the nuclei ( Fig. 2b ). Inhibition of ILK activity also resulted in the interaction of the YAP paralogue, TAZ and 14:3:3 ( Fig. 2c ). Furthermore, inhibition of ILK in several cancer cell lines resulted in the suppression of the transcriptional activity of the TEAD transcription factor ( Fig. 2d ), which is known to be activated by the YAP/TAZ transcriptional co-activators [6] . Since the YAP/TEAD transcription factor complex is known to activate genes involved in cell growth, we determined the effect of the ILK inhibitor on cell growth of PC3 cells. As shown in Fig. 2e , the growth of these cells was significantly inhibited by QLT0267 in a dose-dependent manner. These data demonstrate that ILK suppresses the Hippo pathway in several types of tumour cells through inactivation of the core kinases, MST1, LATS1 and the concomitant activation of YAP/TAZ oncogenes. 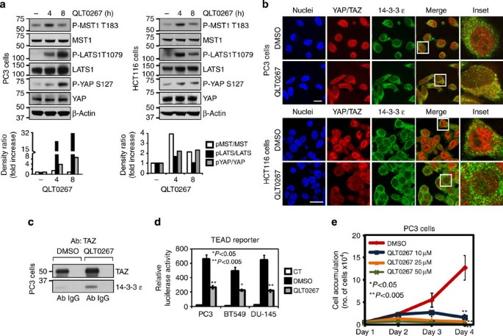Figure 2: Pharmacological inhibition of ILK activates the Hippo pathway and suppresses YAP/TAZ activity in cancer cells. Indicated cells were treated with DMSO (−) or the ILK inhibitor, QLT0267: (a) Cell lysates were subjected to western blotting with the indicated antibodies. Bands were semiquantified by image intensity area under the curve. (b) Cells were subjected to immunofluorescence microscopy with the indicated antibodies. Scale bar, 20 μm. (c) PC3 cells were incubated with DMSO (−) or QLT0267 followed by immunoprecipitation of endogenous TAZ (Ab) or an IgG control (IgG) and subjected to western blot analysis with the indicated antibodies. (d) TEAD transcriptional activity was assessed in the indicated cell lines by TEAD optimal and TEAD inactive mutant (CT)-dependent promoter-driven firefly luciferase reporter construct. Error bars denote s.e.m.P-values were calculated using Student’st-test;n=3 per group. (e) PC3 cells treated with the indicated concentrations of QLT0267 were counted daily to assess cell accumulation. Error bars denote s.e.m.P-values were calculated using Student’st-test;n=3 per group. Figure 2: Pharmacological inhibition of ILK activates the Hippo pathway and suppresses YAP/TAZ activity in cancer cells. Indicated cells were treated with DMSO (−) or the ILK inhibitor, QLT0267: ( a ) Cell lysates were subjected to western blotting with the indicated antibodies. Bands were semiquantified by image intensity area under the curve. ( b ) Cells were subjected to immunofluorescence microscopy with the indicated antibodies. Scale bar, 20 μm. ( c ) PC3 cells were incubated with DMSO (−) or QLT0267 followed by immunoprecipitation of endogenous TAZ (Ab) or an IgG control (IgG) and subjected to western blot analysis with the indicated antibodies. ( d ) TEAD transcriptional activity was assessed in the indicated cell lines by TEAD optimal and TEAD inactive mutant (CT)-dependent promoter-driven firefly luciferase reporter construct. Error bars denote s.e.m. P -values were calculated using Student’s t -test; n =3 per group. ( e ) PC3 cells treated with the indicated concentrations of QLT0267 were counted daily to assess cell accumulation. Error bars denote s.e.m. P -values were calculated using Student’s t -test; n =3 per group. Full size image Growth factor-mediated inactivation of Hippo requires ILK The Hippo pathway has recently been reported to be regulated by G-protein-coupled receptor signalling through lysophosphatidic acid (LPA), as well as by epidermal growth factor (EGF) [13] , [23] . In addition, TGF-β has been shown to activate YAP and YAP-mediated transcription [24] . Since ILK is an established effector of several growth factors, such as TGF-β, EGF, Wnt1 and Wnt3a [16] , [17] , [18] , we wanted to determine whether ILK is required for the suppression of the Hippo pathway and YAP activation by these growth factors. As demonstrated previously, treatment of MCF10A cells with either TGF-β1, EGF or LPA resulted in dephosphorylation of YAP, indicating suppression of Hippo signalling by these factors. However, silencing ILK expression ( Fig. 3a ), inhibited the suppression of phosphorylation of YAP by these factors, thus resulting in stimulation of YAP phosphorylation on Ser127. In addition, nuclear localization of Smad 2/3 was induced in response to TGF-β1 signalling in MCF10A cells independent of ILK as shown previously [16] ( Fig. 3b ). However, TGF-β1-induced nuclear localization of YAP/TAZ was ILK dependent in MCF10A breast and BPH-1 prostate epithelial cells since co-incubation with the ILK inhibitor, QLT0267, or silencing its expression, resulted in the cytoplasmic retention of YAP/TAZ ( Fig. 3b,c ). Interestingly, silencing TAZ and/or YAP expression, resulted in a significant decrease in cell proliferation in MCF10A cells ( Fig. 3d ). The same results in decreased cell proliferation were observed in ILK-depleted cells ( Fig. 3d ). These results suggest that ILK is an upstream regulator of Hippo signalling through multiple growth factor/receptor systems. 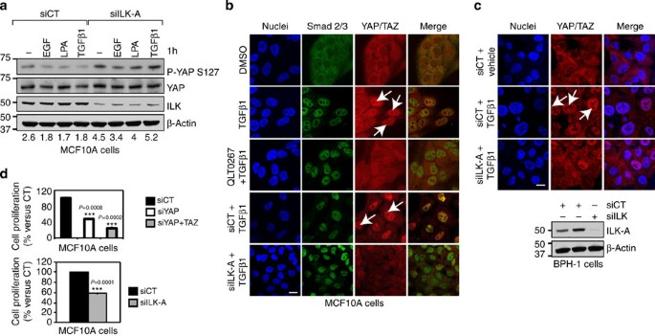Figure 3: ILK is required for growth factor-mediated inactivation of the Hippo pathway. Cells were treated with control (siCT) or ILK (siILK-A) or YAP (siYAP) or TAZ (siTAZ) siRNA, or pretreated with DMSO (−) or QLT0267 for 30 min: (a) Cells were serum-starved and incubated for 1 h with 100 ng ml−1of the indicated growth factors. Cell lysates were subjected to western blotting with the indicated antibodies. Bands were semiquantified by image intensity area under the curve. Numbers represent the ratio of each normalized phospho-Yap band intensity by total-Yap protein band intensity. (b,c) Cells were serum-starved, incubated with 5 ng ml−1TGF-β1 and subjected to immunofluorescence microscopy with the indicated antibodies. Scale bar, 20 μm. ILK depletion by western blot analysis is shown for BPH-1 cells. Arrows indicate nuclear localization. (d) Cell proliferation was assessed by MTT assay. Error bars denote s.e.m.P-values were calculated using Student’st-test;n=3 per group. Figure 3: ILK is required for growth factor-mediated inactivation of the Hippo pathway. Cells were treated with control (siCT) or ILK (siILK-A) or YAP (siYAP) or TAZ (siTAZ) siRNA, or pretreated with DMSO (−) or QLT0267 for 30 min: ( a ) Cells were serum-starved and incubated for 1 h with 100 ng ml −1 of the indicated growth factors. Cell lysates were subjected to western blotting with the indicated antibodies. Bands were semiquantified by image intensity area under the curve. Numbers represent the ratio of each normalized phospho-Yap band intensity by total-Yap protein band intensity. ( b , c ) Cells were serum-starved, incubated with 5 ng ml −1 TGF-β1 and subjected to immunofluorescence microscopy with the indicated antibodies. Scale bar, 20 μm. ILK depletion by western blot analysis is shown for BPH-1 cells. Arrows indicate nuclear localization. ( d ) Cell proliferation was assessed by MTT assay. Error bars denote s.e.m. P -values were calculated using Student’s t -test; n =3 per group. Full size image ILK inhibits Merlin through MYPT1 phosphatase The conserved Hippo pathway is stimulated in mammals by the FERM domain-containing tumour suppressor NF2 (neurofibromatosis type 2)/Merlin, resulting in the sequential activation of the MST1/2 and LATS1/2 kinases [8] . Because the inhibition of ILK in tumour cells significantly enhances the phosphorylation (and thus the activity) of MST1 and LATS1, the point at which ILK affects regulation of the pathway must be upstream of these kinases. Since Merlin is required for MST1 activation [25] , [26] , and Merlin activity is controlled by the phosphorylation status of Ser518 (refs 27 , 28 ), we assessed whether ILK modulates Merlin activation. As shown in Fig. 4a , Merlin was found to be constitutively phosphorylated at its inhibitory site, Ser518 in prostate, colon and breast cancer cells. However, inhibition of ILK activity resulted in dephosphorylation of Merlin Ser518 ( Fig. 4a ). Since Merlin is active when it is dephosphorylated at this site by the myosin phosphatase MYPT1-PP1 (ref. 27) [27] and MYPT1 phosphatase is also an established target of ILK [29] , [30] , we wanted to determine whether ILK might modulate the Hippo pathway through MYPT1-mediated regulation of Merlin phosphorylation. In PC3 cells, MYPT1 was constitutively phosphorylated at its inhibitory site, Thr696 ( Fig. 4b ) [27] , [29] , [30] . However, inhibition of ILK activity resulted in dephosphorylation of MYPT1 ( Fig. 4b ), resulting in its activation as shown previously [29] , [30] , and as determined by the observed dephosphorylation of its target Merlin ( Fig. 4a ). In addition, the activation of the Hippo pathway through inhibition of ILK activity occurred very rapidly as shown by the activation of MYPT1, Merlin and LATS1 in MDA-MB-435 LCC6 cells ( Fig. 4c ). To confirm the specificity of ILK-dependent phosphorylation of MYPT1, especially since MYPT1 can also be phosphorylated at the inhibitory site by Rho kinase [31] , we treated PC3 cells with a Rho kinase-specific inhibitor, H1152. Treatment of PC3 cells with a previously established inhibitory dose of H1152, resulted in only minor inhibition of MYPT1 phosphorylation on Thr696, compared with the effect elicited by QLT0267 ( Fig. 4d ). Consistent with this minor effect on MYPT1 phosphorylation, neither Merlin Ser518 nor LATS1 Thr1079 phosphorylation, were modulated by the Rho kinase inhibitor ( Fig. 4d ). Significantly, only QLT0267, but not H1152, inhibited TEAD transcriptional activity in PC3 cells ( Fig. 4e ). Dephosphorylation of MYPT1 and Merlin was also observed upon siRNA-mediated knockdown of ILK expression in prostate and breast tumour cell lines ( Fig. 4f ). 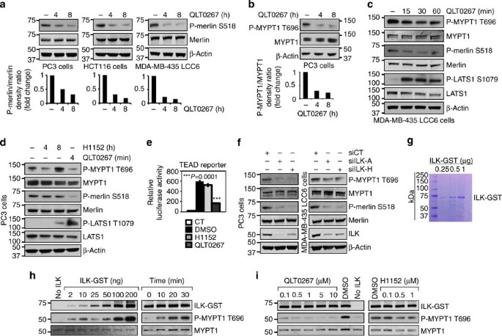Figure 4: ILK inhibits the Hippo pathway through inactivation of Merlin by direct phosphorylation of MYPT1 phosphatase. (a) Indicated cells were treated with DMSO (−) or ILK inhibitor, QLT0267, for the indicated periods of time. Cell lysates were analysed for phospho-Merlin expression by western blotting. Bands were semiquantified by image intensity area under the curve. (b) PC3 cells were treated as described above and analysed for phospho-MYPT1 expression by western blotting. Bands were semiquantified by image intensity area under the curve. (c) MDA-MB-435 LCC6 cells were incubated with DMSO (−) or QLT0267 and subjected to western blot analysis with the indicated antibodies.(d) Indicated cells were treated with DMSO (−), ILK inhibitor, QLT0267 or ROCK inhibitor, H1152, for the indicated periods of time. Hippo pathway components were analysed by western blotting using the indicated antibodies. (e) TEAD transcriptional activity was assessed by TEAD optimal and TEAD inactive mutant (CT)-dependent promoter-driven firefly luciferase reporter construct. Error bars denote s.e.m.P-values were calculated using Student’st-test;n=3 per group. (f) Indicated cells were treated with non-silencing control (siCT) or two different siRNAs against ILK (siILK-A or siILK-H) and cell lysates were subjected to western blotting with the indicated antibodies. (g) The indicated concentrations of GST-ILK were separated by SDS–polyacrylamide gel electrophoresis and subjected to Coomassie blue staining. (h) Western blot analysis of ILK phosphorylation of MYPT1 using various concentrations of ILK-GST (left panel) or reaction incubation times (right panel). Reactions carried out in the absence of GST-ILK are provided as negative controls. (i) Western blot analysis with the indicated antibodies assessing the kinase activity of ILK-GST towards MYPT1 with the indicated concentrations of QLT0267 inhibitor (left panel) or H1152 inhibitor (right panel). Figure 4: ILK inhibits the Hippo pathway through inactivation of Merlin by direct phosphorylation of MYPT1 phosphatase. ( a ) Indicated cells were treated with DMSO (−) or ILK inhibitor, QLT0267, for the indicated periods of time. Cell lysates were analysed for phospho-Merlin expression by western blotting. Bands were semiquantified by image intensity area under the curve. ( b ) PC3 cells were treated as described above and analysed for phospho-MYPT1 expression by western blotting. Bands were semiquantified by image intensity area under the curve. ( c ) MDA-MB-435 LCC6 cells were incubated with DMSO (−) or QLT0267 and subjected to western blot analysis with the indicated antibodies. ( d ) Indicated cells were treated with DMSO (−), ILK inhibitor, QLT0267 or ROCK inhibitor, H1152, for the indicated periods of time. Hippo pathway components were analysed by western blotting using the indicated antibodies. ( e ) TEAD transcriptional activity was assessed by TEAD optimal and TEAD inactive mutant (CT)-dependent promoter-driven firefly luciferase reporter construct. Error bars denote s.e.m. P -values were calculated using Student’s t -test; n =3 per group. ( f ) Indicated cells were treated with non-silencing control (siCT) or two different siRNAs against ILK (siILK-A or siILK-H) and cell lysates were subjected to western blotting with the indicated antibodies. ( g ) The indicated concentrations of GST-ILK were separated by SDS–polyacrylamide gel electrophoresis and subjected to Coomassie blue staining. ( h ) Western blot analysis of ILK phosphorylation of MYPT1 using various concentrations of ILK-GST (left panel) or reaction incubation times (right panel). Reactions carried out in the absence of GST-ILK are provided as negative controls. ( i ) Western blot analysis with the indicated antibodies assessing the kinase activity of ILK-GST towards MYPT1 with the indicated concentrations of QLT0267 inhibitor (left panel) or H1152 inhibitor (right panel). Full size image To confirm that ILK can directly phosphorylate MYPT1 on Thr696, we carried out an in vitro kinase assay utilizing highly purified active recombinant GST-ILK, which has been previously extensively characterized for its kinase characteristics [32] . As shown in Fig. 4g , separation of the GST-ILK by SDS–polyacrylamide gel electrophoresis and staining of the gel with Coomassie blue showed the presence of a full-length protein with the expected molecular weight of ~78 kDa and purity of 94% as shown previously [32] . In addition, mass spectrometric analysis demonstrated the absence of other protein kinases in the GST-ILK preparation used for these studies [32] . This recombinant ILK directly phosphorylated MYPT1 on the inhibitory Thr696 residue in a dose and time-dependent manner ( Fig. 4h ), and this phosphorylation was inhibited by the ILK inhibitor, QLT0267 ( Fig. 4i ) but not by the Rho kinase inhibitor, H1152 ( Fig. 4i ). These data demonstrate the specificity of ILK in regulating the phosphorylation of MYPT1 at its inhibitory site. Furthermore, we silenced MYPT1 expression in PC3 cells to determine whether MYPT1 is required for the ILK-mediated constitutive phosphorylation and inactivation of Merlin. Treatment of the MYPT1 knockdown cells with QLT0267 did not result in a significant effect on Merlin phosphorylation ( Fig. 5a ). However, the inhibition of Ser473 Akt phosphorylation by QLT0267 was similar in control and MYPT1-silenced cells ( Fig. 5a ), suggesting a specific role of the ILK-MYPT1-Merlin axis in the regulation of the Hippo pathway. Finally, we examined the effect of ILK inhibition in U87 MG human malignant glioma cell line, in which Merlin expression has been shown to be dramatically reduced [33] , and also in Merlin-deficient Meso-33 mesothelioma cells [34] . As shown in Fig. 5b , no differences were observed in YAP/TAZ localization upon treatment of these cell lines with the ILK inhibitor, QLT0267. These data suggest that ILK regulates the Hippo pathway largely through MYPT1/Merlin axis, although, the regulation by ILK of other MST1/LATS1 modulators may also play a role. 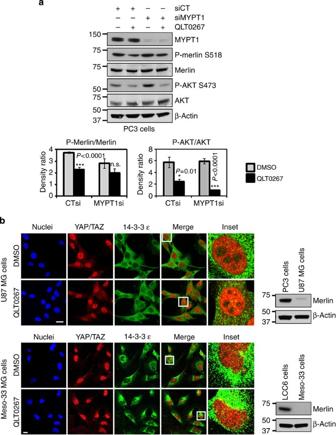Figure 5: ILK requires MYPT1 and Merlin to inactivate the Hippo pathway. (a) PC3 cells were treated with non-silencing control (siCT) or siRNA against MYPT1 (siMYPT1) were incubated with DMSO or ILK inhibitor QLT0267 and cell lysates were subjected to western blotting with the indicated antibodies. Bands were semiquantified by image intensity area under the curve and represented as the ratio of each normalized phospho-antibody band intensity by total protein band intensity. Error bars denote s.e.m.P-values were calculated using Student’st-test;n=4 independent experiments. Not significant (n.s.). (b) Indicated cells were treated with DMSO or the ILK inhibitor QLT0267, fixed and subjected to immunofluorescence microscopy with the indicated antibodies. Scale bar, 20 μm. Right panels show Merlin expression in comparison with other cell lines by western blot analysis. Figure 5: ILK requires MYPT1 and Merlin to inactivate the Hippo pathway. ( a ) PC3 cells were treated with non-silencing control (siCT) or siRNA against MYPT1 (siMYPT1) were incubated with DMSO or ILK inhibitor QLT0267 and cell lysates were subjected to western blotting with the indicated antibodies. Bands were semiquantified by image intensity area under the curve and represented as the ratio of each normalized phospho-antibody band intensity by total protein band intensity. Error bars denote s.e.m. P -values were calculated using Student’s t -test; n =4 independent experiments. Not significant (n.s.). ( b ) Indicated cells were treated with DMSO or the ILK inhibitor QLT0267, fixed and subjected to immunofluorescence microscopy with the indicated antibodies. Scale bar, 20 μm. Right panels show Merlin expression in comparison with other cell lines by western blot analysis. Full size image YAP and TAZ activation is ILK dependent in tumours in vivo In order to determine whether the role of ILK in suppressing the Hippo pathway extended to tumours in vivo , we took advantage of two previously established transgenic breast cancer models in which the ILK gene was either deleted from ErbB2-induced breast tumours [35] , or was overexpressed together with Wnt1 in the mammary epithelium [36] . In the former case deletion of ILK had a significant growth suppressive and anti-metastatic effect on ErbB2-driven mammary tumours [35] , whereas breast tumour growth in the double-transgenic Wnt1/ILK mice was significantly accelerated largely due to more rapid cell proliferation [36] . Here we now show that YAP/TAZ is highly expressed in ErbB2-driven mammary tumours ( Fig. 6a ) with a significant proportion of its expression within the nuclei of the tumour cells. Deletion of ILK in the background of ErbB2 activation resulted in dramatic inhibition of YAP/TAZ expression ( Fig. 6a ), and silencing ILK in cell lines established from the ErbB2 tumours resulted in sequestration of YAP in the cytoplasm as well as in the inhibition of TEAD reporter activity ( Fig. 6b,c ), demonstrating that ErbB2-driven YAP expression requires ILK. The converse was observed in the tumours derived from the Wnt1/ILK double-transgenic mice relative to tumours derived from the single Wnt1 mice. Nuclear YAP expression was significantly elevated in the double-transgenic tumours compared with the Wnt1 only tumours ( Fig. 6d ), suggesting that YAP expression can be co-operatively driven by Wnt and ILK. These in vivo tumour models, where expression of ILK has been altered chronically, demonstrate that YAP/TAZ activation, and therefore accumulation, depend on ILK. 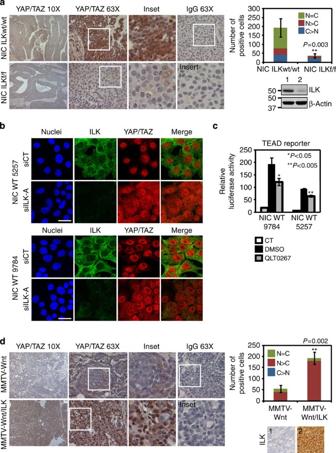Figure 6: ILK inactivates the Hippo tumour suppressor pathwayin vivo. (a) Immunohistochemistry analysis of ErbB2-induced tumours with YAP/TAZ or an IgG control (IgG) antibody. Number of cells with nuclear and cytoplasmic (green,n=C), predominantly nuclear (red, N>C) and predominantly cytoplasmic (blue, C>N) YAP/TAZ localization were quantified in random 63 × views (right panel). Error bars denote s.e.m.P-values were calculated using Student’st-test;n=5 tumours per group. Lysates from tumours were subjected to western blotting to determine ILK expression (bottom right panel; 1=ILKwt/wt, 2=ILKf/f). (b,c) NIC WT cell lines established from the ErbB2 tumours were (b) treated with non-silencing control (siCT) or ILK siRNA (siILK-A), and subjected to immunofluorescence microscopy with the indicated antibodies. Scale bar, 20 μm. Or (c) treated with DMSO or ILK inhibitor QLT0267 and TEAD transcriptional activity was assessed by TEAD optimal and TEAD inactive mutant (CT)-dependent promoter-driven firefly luciferase reporter construct. Error bars denote s.e.m.P-values were calculated using Student’st-test;n=3 per group. (d) Immunohistochemistry analysis of Wnt1- and double-transgenic Wnt1/ILK-derived tumours with YAP/TAZ or an IgG control (IgG) antibody or ILK (1=Wnt, 2=Wnt/ILK). Number of cells with nuclear and cytoplasmic (green,n=C), predominantly nuclear (red, N>C) and predominantly cytoplasmic (blue, C>N) YAP/TAZ localization were quantified in random 63 × views (right panel). Error bars denote s.e.m.P-values were calculated using Student’st-test;n=4 tumours per group. Figure 6: ILK inactivates the Hippo tumour suppressor pathway in vivo . ( a ) Immunohistochemistry analysis of ErbB2-induced tumours with YAP/TAZ or an IgG control (IgG) antibody. Number of cells with nuclear and cytoplasmic (green, n =C), predominantly nuclear (red, N>C) and predominantly cytoplasmic (blue, C>N) YAP/TAZ localization were quantified in random 63 × views (right panel). Error bars denote s.e.m. P -values were calculated using Student’s t -test; n =5 tumours per group. Lysates from tumours were subjected to western blotting to determine ILK expression (bottom right panel; 1=ILKwt/wt, 2=ILKf/f). ( b , c ) NIC WT cell lines established from the ErbB2 tumours were ( b ) treated with non-silencing control (siCT) or ILK siRNA (siILK-A), and subjected to immunofluorescence microscopy with the indicated antibodies. Scale bar, 20 μm. Or ( c ) treated with DMSO or ILK inhibitor QLT0267 and TEAD transcriptional activity was assessed by TEAD optimal and TEAD inactive mutant (CT)-dependent promoter-driven firefly luciferase reporter construct. Error bars denote s.e.m. P -values were calculated using Student’s t -test; n =3 per group. ( d ) Immunohistochemistry analysis of Wnt1- and double-transgenic Wnt1/ILK-derived tumours with YAP/TAZ or an IgG control (IgG) antibody or ILK (1=Wnt, 2=Wnt/ILK). Number of cells with nuclear and cytoplasmic (green, n =C), predominantly nuclear (red, N>C) and predominantly cytoplasmic (blue, C>N) YAP/TAZ localization were quantified in random 63 × views (right panel). Error bars denote s.e.m. P -values were calculated using Student’s t -test; n =4 tumours per group. Full size image Inhibition of ILK in vivo results in decreased tumour growth We next sought to characterize the efficacy of ILK inhibition with QLT0267 in vivo . We used MDA-MB-435 LCC6 cells, an established xenograft model for evaluating the efficacy of anti-cancer agents [37] , to first demonstrate the inhibition of TEAD transcriptional activity, induction of apoptosis and reduced cell growth in vitro following QLT0267 treatment ( Fig. 7a–c ). ILK may promote cell growth and survival through activation of different signalling pathways such as PI3K/Akt [17] . To assess whether the induction of apoptosis and reduced cell growth observed following QLT0267 treatment in MDA-MB-435 cells was dependent on the inactivation of YAP/TAZ oncogenes, cells were transfected with an activated form of YAP (YAP S127A) [12] . Transfection of YAP S127A in MDA-MB-435 LCC6 cells prior to incubation with the ILK inhibitor QLT0267, resulted in a nearly complete rescue of apoptosis ( Fig. 7d ) and to partial rescue of cell growth inhibition ( Fig. 7e ). These results demonstrate that ILK promotes cell growth and survival of these cells at least partially through inactivation of the Hippo pathway. Finally, treatment of mice with established tumours derived from these cells with QLT0267 resulted in significant tumour growth suppression ( Fig. 7f ) while simultaneously resulting in the inhibition of expression of nuclear YAP in the tumour cells within the tumours ( Fig. 7g ). A caveat of the effects of QLT0267 on tumour growth and YAP expression in mice could be through potential off-target effects due to the inhibition of other protein kinases as shown by Eke et al. [38] In conclusion, we have identified ILK as a critical player in the inactivation of the Hippo tumour suppressor pathway, via inactivation of the tumour suppressor Merlin. Importantly, we show that inhibition of ILK can switch the Hippo pathway ‘on’, resulting in the inactivation of YAP/TAZ and TEAD transcriptional activity, inhibition of tumour cell growth, induction of apoptosis and suppression of tumour growth in vivo ( Fig. 8 ). 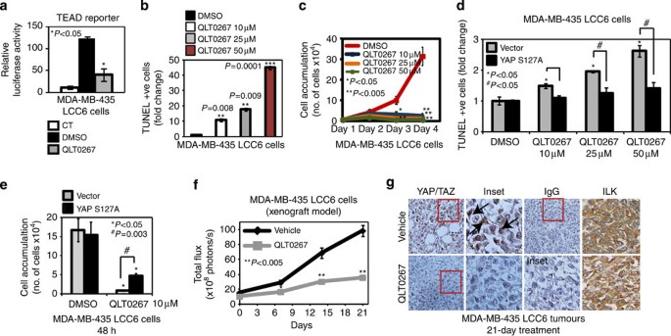Figure 7: Pharmacological inhibition of ILKin vivoleads to decreased tumour growth and YAP/TAZ inactivation. (a–e) Cells were treated with DMSO or ILK inhibitor QLT0267 at indicated concentrations: (a) TEAD transcriptional activity was assayed using TEAD optimal and TEAD inactive mutant (CT)-dependent promoter-driven firefly luciferase reporter construct. Error bars denote s.e.m.P-values were calculated using Student’st-test;n=3 per group. (b) Apoptosis was measured by TUNEL. Error bars denote s.e.m.P-values were calculated using Student’st-test;n=3 per group. (c) Cells were counted daily to assess cell accumulation. Error bars denote s.e.m.P-values were calculated using Student’st-test;n=3 per group. (d,e) Prior to treatment, cells were transfected with vector or constitutive active YAP (YAP S127A): (d) Apoptosis was measured by TUNEL. Error bars denote s.e.m.P-values were calculated using Student’st-test;n=3 per group. (e) Cells were counted daily to assess cell accumulation. Error bars denote s.e.m.P-values were calculated using Student’st-test;n=3 per group. (f) Luciferase-labelled MDA-MB-435 LCC6 cells were implanted orthotopically into Balb/c mice and treatment (Tx) was initiated 1 week later. Vehicle or 200 mg kg−1QLT0267 were administered daily by oral gavage and tumour growth was monitored by IVIS imaging. Error bars denote s.e.m.P-values were calculated using Student’st-test;n=10–16 mice per group. (g) At the end of treatment, tumours were excised and subjected to immunohistochemistry with YAP/TAZ, or IgG control (IgG), or ILK antibodies. Representative images are shown. Arrows indicate YAP/TAZ nuclear localization. YAP/TAZ and IgG original magnifications × 63, ILK original magnification × 40. Figure 7: Pharmacological inhibition of ILK in vivo leads to decreased tumour growth and YAP/TAZ inactivation. ( a – e ) Cells were treated with DMSO or ILK inhibitor QLT0267 at indicated concentrations: ( a ) TEAD transcriptional activity was assayed using TEAD optimal and TEAD inactive mutant (CT)-dependent promoter-driven firefly luciferase reporter construct. Error bars denote s.e.m. P -values were calculated using Student’s t -test; n =3 per group. ( b ) Apoptosis was measured by TUNEL. Error bars denote s.e.m. P -values were calculated using Student’s t -test; n =3 per group. ( c ) Cells were counted daily to assess cell accumulation. Error bars denote s.e.m. P -values were calculated using Student’s t -test; n =3 per group. ( d , e ) Prior to treatment, cells were transfected with vector or constitutive active YAP (YAP S127A): ( d ) Apoptosis was measured by TUNEL. Error bars denote s.e.m. P -values were calculated using Student’s t -test; n =3 per group. ( e ) Cells were counted daily to assess cell accumulation. Error bars denote s.e.m. P -values were calculated using Student’s t -test; n =3 per group. ( f ) Luciferase-labelled MDA-MB-435 LCC6 cells were implanted orthotopically into Balb/c mice and treatment (Tx) was initiated 1 week later. Vehicle or 200 mg kg −1 QLT0267 were administered daily by oral gavage and tumour growth was monitored by IVIS imaging. Error bars denote s.e.m. P -values were calculated using Student’s t -test; n =10–16 mice per group. ( g ) At the end of treatment, tumours were excised and subjected to immunohistochemistry with YAP/TAZ, or IgG control (IgG), or ILK antibodies. Representative images are shown. Arrows indicate YAP/TAZ nuclear localization. YAP/TAZ and IgG original magnifications × 63, ILK original magnification × 40. 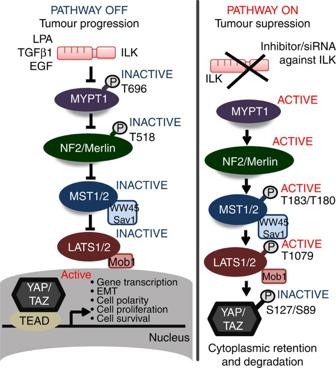Figure 8: Model for ILK regulation of the Hippo pathway. PATHWAY OFF: ILK promotes tumour progression through phospho-dependent inactivation of MYPT1 phosphatase leading to inactivation of Merlin/MST/LATS key components of the Hippo pathway. PATHWAY ON: inhibition or genetic depletion of ILK results in the activation of the Hippo pathway resulting in the cytoplasmic retention and degradation of YAP/TAZ oncogenes and inhibition of tumour growth. Full size image Figure 8: Model for ILK regulation of the Hippo pathway. PATHWAY OFF: ILK promotes tumour progression through phospho-dependent inactivation of MYPT1 phosphatase leading to inactivation of Merlin/MST/LATS key components of the Hippo pathway. PATHWAY ON: inhibition or genetic depletion of ILK results in the activation of the Hippo pathway resulting in the cytoplasmic retention and degradation of YAP/TAZ oncogenes and inhibition of tumour growth. Full size image The communication between cells and their microenvironment can influence activation or inactivation of intracellular signalling pathways and the survival of tumour cells depends on their ability to adapt to their environment [3] , [4] , [6] . Integration of signalling pathways for the adequate balance of cell proliferation and apoptosis is an essential function of multicellular organism under physiological conditions and deregulation of these functions leads to human diseases such as cancer. The Hippo tumour suppressor pathway plays an important role in the maintenance of this cell number balance, and its deregulation promotes tumorigenesis. Although the transcription co-activators, YAP and TAZ, are well-established Hippo signalling downstream oncogenes in several cell types and promote metastasis [6] , [12] , [25] , [39] , many efforts are now directed towards identifying the upstream regulators of the pathway. Other kinases such as homeodomain-interacting protein kinase (HIPK2) have been recently identified to modulate YAP [40] . However, in contrast to ILK, which we have demonstrated is upstream of LATS phosphorylation and activation, regulation of YAP by HIPK2 occurs in parallel to LATS activation [40] . In the context of normal hepatic biology and control of organ size, it has been reported that targeted knockout of ILK in the liver results in increased expression of total YAP during liver regeneration [41] . Overall lower phosphorylation of YAP in the knockout animals was also reported in this study, although results were not quantified and other components of the Hippo pathway were not interrogated [41] . Importantly, we have demonstrated in this study that ILK is a critical upstream regulator of Hippo signalling in cancer cells and that inhibition of ILK leads to changes in the phosphorylation status of several of the core components of the pathway (MST1, LATS1 and YAP), resulting in the inactivation of YAP. Thus, our data suggest a novel mechanism of regulation of the Hippo pathway by ILK in tumour cells. The differences between the data described here and those reported by Apte et al. [41] may be due, in part, to the contrasting roles of ILK signalling in normal cells and cancer cells, as has been established previously for the survival of cancer cells, which are critically dependent on ILK signalling, compared with ILK-independent survival by normal cells [21] . We have shown that the Hippo tumour suppressor pathway is inactivated in human breast, prostate and colon cancer cell lines, as indicated by the low or undetectable phosphorylation of MST1, LATS1 and YAP proteins, YAP/TAZ nuclear localization and high TEAD transcriptional activity. Inhibition of ILK activity or siRNA-mediated silencing of its expression resulted in a complete reversal of the pathway. Merlin, the product of NF2 gene, serves as a linker between transmembrane proteins and the actin cytoskeleton. Merlin is a multifunctional protein and recent studies suggest that Merlin is also an upstream component of the mammalian Hippo pathway [26] , [42] , [43] , [44] . Our results demonstrate that in the tumour cell types in which the Hippo pathway is inactivated, Merlin is phosphorylated on Ser518. Inhibiting or silencing ILK resulted in dephosphorylation of Merlin at this site, and since activation of Merlin occurs upon its dephosphorylation [27] , ILK most likely regulates Merlin phosphorylation via phospho-inhibition of a phosphatase. It has been shown that Merlin is the decisive substrate of MYPT1-PP1 in tumour suppression [27] and here we have demonstrated that ILK specifically phosphorylates MYPT1 to inhibit its activity. The GST-ILK preparation used to perform the kinase assay experiments reported in this study has been extensively characterized [32] . In fact, mass spectrometric analysis of the highly purified preparation did not detect any other protein kinases, besides ILK [32] , demonstrating that ILK alone is responsible for MYPT1 phosphorylation in this assay. Furthermore, inhibition of ILK in MYPT1-depleted cells or Merlin-deficient cells did not have any effect on the downstream components of the pathway, demonstrating that MYPT1 and Merlin are required for the regulation of the pathway by ILK. Importantly, our data demonstrating that YAP/TAZ inactivation in cancer cells in response to genetic silencing of ILK expression using two independently targeted siRNA sequences correlates with the results of pharmacologic inhibition of ILK activity using a well-established, selective ILK inhibitor in the same cell types, together with our results showing that MYPT1 is directly phosphorylated by purified ILK in vitro and that this phosphorylation is inhibited by QLT0267, but not by a Rho kinase inhibitor, constitute further convincing evidence that ILK is an active, physiologically relevant kinase [45] . Recently, numerous upstream components involved in the Hippo pathway have been identified, such as cell polarity, mechanotransduction and G-protein-coupled receptor signalling [44] , [46] , and Hippo signalling has been shown to be regulated by cell detachment and by growth factors [13] , [14] . We found that the suppression of the Hippo pathway by the tumour microenvironmental factors TGF-β, EGF and LPA is ILK dependent. These results suggest that the regulation of the Hippo pathway by ILK is through multiple growth factors signalling receptor. Both ILK and YAP/TAZ protein levels are frequently elevated in many types of human cancers [17] , [25] , [47] , [48] , [49] , although whether these elevated levels interact functionally has not been determined. Here, we have provided compelling evidence for such a functional interaction between ILK and activation of YAP/TAZ in cancer cell lines and in breast tumours in vivo . First, in ErbB2-induced mammary tumours, where YAP/TAZ are highly expressed and active, deletion of ILK had a significant suppression of YAP/TAZ expression, correlating with a marked suppression of tumour growth and metastasis [35] . The overall decrease in YAP protein expression in the ILK knockout tumours is somewhat different from what we observed with ILK knockdown or inhibition of activity in cultured cells where the overall levels of YAP/TAZ were not suppressed, but rather they were sequestered in the cytoplasm. The overall decrease in the YAP/TAZ protein levels in these tumours in vivo is not surprising however, since YAP/TAZ phosphorylation also leads to its degradation [49] , and long-term sequestration in the cytoplasm would also lead to eventual degradation. Recently, coordinated phosphorylation of YAP by LATS and CK1 on Ser381 has been shown to regulate the stability of YAP [50] , and this could account for the loss of YAP expression in the ILK knockout tumours. Second, we have shown the converse situation where tumours that overexpress ILK in the background of Wnt activation leads to accelerated tumour growth [36] and have increased and strong nuclear expression of YAP/TAZ proteins. Wnt signalling is known to activate the expression of YAP/TAZ [51] , and β-catenin-driven cancers require YAP transcriptional complex for tumorigenesis [52] . Since ILK also activates the downstream components of the Wnt signalling pathway, especially β-catenin stabilization [53] , and it cooperates with Wnt1 to accelerate breast tumour growth [36] , it is not surprising to observe significant stimulation of nuclear YAP expression in tumours from the double-transgenic ILK/Wnt1 mice. These data suggest that ILK can also regulate YAP/TAZ in a Hippo pathway-independent manner. Third, treatment with QLT0267 in MDA-MB-435 LCC6 established xenograft model for evaluating the efficacy of anti-cancer agents [37] , resulted in significant tumour growth suppression with inhibition of expression of nuclear YAP/TAZ in the tumour cells within the tumours. Collectively, these data suggest that YAP/TAZ activation can be driven by ILK in vivo . The Hippo pathway plays a critical role in tumour growth and metastasis and pharmacological interventions of this pathway have important clinical implications. With this work, we have provided new insights into the regulation of this tumour suppressor pathway, demonstrating that ILK is a negative regulator of the Hippo pathway and we have provided data suggesting that ILK is a potential therapeutic target, the inhibition of which can activate the Hippo kinase cascade to inactivate YAP/TAZ oncogenes and inhibit tumour cell growth. Cell culture and transfection Human breast cancer cells (MDA-MB-231, MDA-MB-435 LCC6 and BT549), prostate cancer cells (PC3 and DU-145), U87 MG glioma cells and normal prostate BPH-1 cells were originally obtained from the American Type Culture Collection (ATCC, Manassas, VA) and were cultured in high-glucose DMEM (Invitrogen, Canada) with 2 mmol l −1 L -glutamine and 10% fetal bovine serum (Invitrogen). Normal human epithelial MCF10A cells were cultured as previously described [12] , [16] . NIC wild-type (WT) 9784 and 5257, were isolated from ErbB2-induced mammary tumours (NIC ILK wt/wt) and grown in DMEM with 5% fetal bovine serum, EGF (5 ng ml −1 , Sigma-Aldrich), hydrocortisone (1 μg ml −1 , Sigma-Aldrich), insulin (5 μg ml −1 , Sigma-Aldrich) and bovine pituitary extract (Lonza) [35] . Meso-33 cells were a gift from Dr Filippo G. Giancotti (Memorial Sloan-Kettering Cancer Center (MSKCC), New York, NY, USA). Cells were incubated with the ILK inhibitor, 10 μM QLT0267 (unless otherwise specified) (Quadralogic Technologies Inc, Vancouver, BC, Canada) or the Rho kinase inhibitor, 1 μM H1152 (Millipore), at times specified in the text and control cells were incubated with DMSO vehicle (Sigma-Aldrich). For siRNA (small interference) transfection, cells were transfected using SilentFect (Bio-Rad Laboratories) as previously shown [16] . ILK was targeted, as previously validated [16] , [54] , using ILK-A, DNA target sequence: AAGACGCTCAGCAGACATGTGGA or ILK-H, DNA target sequence: AACCTGACGAAGCTCAACGAG. siRNA against YAP (cat. no. sc-38637), TAZ (cat. no. sc-38568) and MYPT1 (cat. no. sc-37240) were purchased from Santa Cruz. For vector and YAP S127A DNA transfection, cells were transfected using Lipofectamine 2000 (Invitrogen) according to manufacturer’s instructions. Luciferase assay For TEAD transcriptional activity assays, the indicated cells were plated on 24-well dishes in triplicates and co-transfected with 400 ng of a 20:1 mixture of 10 × optimal TEAD BS in pGL3-Basic or 10 × mutant TEAD BS in pGL3-Basic as a control (CT) and PRL-TK using Lipofectamine Plus (Invitrogen). After 48 h, cells were treated overnight with DMSO or 10 μM QLT0267 and luciferase activity was assayed using the dual luciferase reporter assay system (Promega) and the Lumat LB 9507 plate reader. For each triplicate well the signal of firefly luciferase (pGL3-10 × Basic) was normalized to the signal for Renilla luciferase (PRL-TK). Growth factors MCF10A cells were serum-starved overnight and incubated with 10% horse serum or 100 ng ml −1 of EGF (Sigma-Aldrich), L -a-LPA (Sigma-Aldrich) or TGF-β1 (R&D Systems, Canada). Cells were previously treated with DMSO or 10 μM QLT0267 for 30 min or ILK silenced using siRNA. For YAP/TAZ immunofluorescence localization experiments, MCF10A or BPH-1 cells were serum-starved and incubated with 5 ng ml −1 human recombinant TGF-β1 (R&D Systems, Canada) or vehicle (4 mM HCl containing 1 mg ml −1 bovine serum albumin) for 2 h. Co-incubation with DMSO or 10 μM QLT0267 was also carried out as appropriate or ILK expression was silenced using siRNA. Cell proliferation and apoptosis assays Indicated cells were maintained in the presence or absence of 10, 25 or 50 μM QLT0267 for 1, 2 or 3 days. For cell proliferation, cell numbers were determined daily using a cell counter (Bio-Rad) or as for MCF10A cells, Cell Proliferation Kit I (MTT) was used following the manufacturer’s instructions (Roche). To assess cell apoptosis, cells were incubated with the inhibitor at indicated concentrations for 24 h, fixed with 4% paraformaldehyde, permeabilized with 0.2% Triton-x-100 (Sigma-Aldrich) and subjected to TUNEL protocol using In Situ Cell Death Detection Kit (Roche Diagnostics) following the manufacturer’s instructions. DNase I-treated (Invitrogen) sections and sections incubated with label solution only, were used for positive and negative controls, respectively. Cell lysis and immunoprecipitation Cells were harvested and RIPA lysed as described previously [16] . For immunoprecipitation experiments, cells were pelleted and resuspended in 400 μl of 10 mM HEPES-potassium hydroxide (pH 7.9), 1.5 mM magnesium chloride, 10 mM potassium chloride, 0.5 mM dithiothreitol and 0.2 mM phenylmethylsulphonyl fluoride. After 10 min of incubation on ice, nuclei were pelleted by being spun for 10 s and resuspended in 50 μl of 20 mM HEPES-potassium hydroxide (pH 7.9), 25% glycerol, 420 mM sodium chloride, 1.5 mM magnesium chloride, 0.2 mM EDTA, 0.5 mM dithiothreitol and 0.2 mM phenylmethylsulphonyl fluoride. Tubes were incubated for 20 min on ice and then centrifuged to clear the cellular debris [53] . Protein concentrations were determined using the BCA assay (Pierce Biotechnology). Immunoprecipitation of 1 mg protein was carried in the cytoplasmic cell fraction with 5 μg anti-TAZ antibody (cat. no. 560235, BD Bioscience) or the correspondent mouse IgG control antibody (sc-2025, Santa Cruz). Western blotting Immunoblotting was carried out as previously described [16] . Proteins were separated on NuPAGE 4–12% gradient gels (Invitrogen). Samples were incubated overnight at 4 °C with appropriate primary antibodies at a dilution of 1:1,000: anti-phospho-LATS1 Thr1079 (cat. no. 9159), anti-LATS1 (cat. no. 3477), anti-phospho-MST1 Thr183/Mst2 Thr180 (cat. no. 3681), anti-phospho-Merlin Ser518 (cat. no. 9163), anti-phospho-YAP Ser127 (cat. no. 4911), anti-MYPT1 (cat. no. 2634), anti-YAP/TAZ (cat. no. 8418) (Cell Signaling), anti-MST1 (cat. no. ab57836), anti-NF2/Merlin (cat. no. ab88957), anti-14:3:3 ε (cat. no. 92311) (Abcam), anti-ILK (cat. no. 611803, BD Transductions), anti-β-actin (cat. no. A5441, Sigma-Aldrich), anti-YAP (sc-101199) and anti-phospho-MYPT1 Thr696 (ABS45, Millipore). Proteins were visualized by chemiluminescence (ECL or supersignal, Pierce) or using the Odyssey system (Li-Cor Biosciences). Densitometric analysis of the blots was performed using ImageJ software (National Institutes of Health, USA). Full blots can be found in Supplementary Figs S1–S6 . Quantification of western blots Bands were semiquantified by image intensity under the curve. For phospho-protein levels, the ratio of the intensity of the phospho-protein band to the total protein band in each lane was calculated. For ILK protein levels, the ratio of ILK to β-actin was calculated. For data presented as bar graphs, control samples were set at 1 and fold change in intensity is reported. For data presented as values directly below the blots, the ratio of phospho-protein to total protein is reported. Data are representative of at least three independent experiments. Immunofluorescence microscopy Cells were treated with the indicated inhibitors for 2 h, washed with PBS, fixed with 4% paraformaldehyde and permeabilized with 0.2% Triton-x-100 (Sigma-Aldrich). Primary antibodies: anti-ILK (cat. no. 611803, 1:100), anti-Smad 2/3 (cat. no. 610842, 1:100) (BD Transduction), anti-YAP/TAZ (cat. no. 8418, Cell Signaling, 1:50) and anti-14:3:3 ε (sc-135816, Santa Cruz, 1:50) were used followed by the appropriate anti-mouse or anti-rabbit Alexa Fluor 488 and 594 secondary antibodies (Invitrogen). Nuclei were stained using bisBenzimide Hoescht 33342 trihydrochloride (Sigma-Aldrich). Samples were mounted using Mowiol 4–88 (Polysciences). Images were taken using Zeiss 780 confocal microscope. Representative images of at least three independent experiments are shown. Areas indicated with a square box were cropped for more detail in the figures (inset, Fig. 1b , 2b , 5b , 6a, 6d and 7g ). Kinase activity assay Non-radioactive ILK kinase activity assays were performed as previously described [32] . Briefly, 100 ng of highly purified GST-ILK (SignalChem Lifesciences Corporation, Richmond, BC, Canada), 500 ng of the substrate MYPT1 (EMD Millipore, Billerica, MA) and 500 μM cold ATP were incubated in kinase buffer (New England Biolabs, Ipswich, MA) in a total volume of 20 μl. Reactions were carried out at 30 °C for 30 min in a circulating water bath. For experiments using kinase inhibitors, stock inhibitors in DMSO were initially diluted in water to create working stocks. One microlitre volumes of the inhibitor working stocks were added directly to the kinase reaction to provide final inhibitor concentrations as indicated in the figures. Inhibitors included Rho kinase inhibitor (EMD Millipore) and ILK kinase inhibitor QLT0267 (Quadralogic Technologies Inc., Vancouver, BC, Canada). Transgenic mouse models and immunohistochemistry ErbB2-induced mammary tumours (NIC ILK wt/wt) or mammary gland targeted deletion of ILK tumours (NIC ILK f/f) have been generated and characterized [35] . To mitigate the impact of genetic background variability, transgenic mice were derived from the inbred FVB/N strain. Mammary tumour formation was monitored by weekly palpations. The generation of mammary-specific double-transgenic MMTV-Wnt/ILK mice has been described by us [36] . Briefly, MMTV-Wnt1 and MMTV-ILK mice were backcrossed to the FVB strain. MMTV-Wnt1 males were then bred with MMTV-ILK female to generate the double-transgenic MMTV-Wnt/ILK mice. Mice were tail clipped and genotyped by PCR. Nulliparous females were monitored biweekly for tumours by palpation and tumour growth was monitored by caliper measurement subsequent to tumour discovery. All tumour samples were fixed in 10% neutral-buffered formalin, paraffin-embedded and sectioned at 4 μm. Immunohistochemistry analysis was performed as previously described [35] , [55] . Briefly, antigen retrieval was accomplished in citrate buffer by using a microwave and peroxidase activity was blocked with 3% peroxide hydrogen. Sections were then blocked in 5% goat serum or milk and incubated in primary antibodies (1:100 dilution) anti-YAP/TAZ (cat. no. 8418, Cell Signaling) or anti-ILK (sc-20019, Santa Cruz). Areas indicated with a square box were cropped for more detail (inset). Human breast cancer xenografts All animal studies and procedures were performed in accordance with protocols approved by the Animal Care Committee at the University of British Columbia and the BC Cancer Research Centre-BC Cancer Agency. MDA-MB-435/LCC6 GFP/Luc cells were inoculated into the mammary fat pad of a 7–10-week-old female Rag-2M mice. Tumours were allowed to establish for 7 days. Caliper measurements were initiated ~5–7 days post cell inoculation, when tumours become palpable by hand were visible, and were conducted once per week. Vehicle PTE (PEG300/Ethanol/Tween 80/citrate (63:29:7.8:0.2 w/v/w/w)) or QLT0267 (200, 150 or 75 mg kg −1 ) were administered daily by oral gavage. Tumour growth was monitored by IVIS imaging for luciferase-labelled MDA-MB-435/LCC6 GFP/Luc cells. Tumours were excised at days indicated in the text and paraffin-embedded for immunohistological staining. Statistical analysis With the exception of western blot analysis (described above), graphical data are presented as mean values±standard error (s.e.m.). P -values were calculated using unpaired Student’s t -tests comparing control with treated cells/animals. Statistically significant differences are indicated within the text and by asterisks. Data are representative of at least three independent experiments. How to cite this article : Serrano, I. et al. Inactivation of the Hippo tumour suppressor pathway by integrin-linked kinase. Nat. Commun. 4:2976 doi: 10.1038/ncomms3976 (2013).